Reward-timing-dependent bidirectional modulation of cortical microcircuits during optical single-neuron operant conditioning Animals rapidly adapt to environmental change. To reveal how cortical microcircuits are rapidly reorganized when an animal recognizes novel reward contingency, we conduct two-photon calcium imaging of layer 2/3 motor cortex neurons in mice and simultaneously reinforce the activity of a single cortical neuron with water delivery. Here we show that when the target neuron is not relevant to a pre-trained forelimb movement, the mouse increases the target neuron activity and the number of rewards delivered during 15-min operant conditioning without changing forelimb movement behaviour. The reinforcement bidirectionally modulates the activity of subsets of non-target neurons, independent of distance from the target neuron. The bidirectional modulation depends on the relative timing between the reward delivery and the neuronal activity, and is recreated by pairing reward delivery and photoactivation of a subset of neurons. Reward-timing-dependent bidirectional modulation may be one of the fundamental processes in microcircuit reorganization for rapid adaptation. Animals can rapidly adapt to environmental changes. This is accomplished by the reorganization of neuronal activity. When the adaptation requires body movement, activity changes occur in many motor cortex neurons associated with motor commands and proprioceptive feedback [1] . By contrast, when the adaptation does not require body movement and the cortical activity is reinforced with repeated reward deliveries, primates can volitionally control the cortical activity at the level of single neurons [1] , [2] , [3] , [4] , [5] . Single-neuron operant conditioning (SNOC) provides a framework for studying the reorganization of neuronal activity during rapid adaptation because it is accompanied by modulation of the activity of non-target neurons, and the associations between non-target and target neurons can be unambiguously determined. Theoretically, cortical reorganization during both SNOC and brain-machine and brain-computer interface learning can be explained by reward-timing-dependent plasticity, in which the activity change in an individual neuron depends on the activity timing relative to a global reward signal [6] , [7] , [8] . In addition to the inputs associated with the global reward signal, cortical neurons receive strong synaptic inputs from surrounding neurons. Consistent with this, non-target neurons whose activity is highly correlated with that of the target neuron tend to change their firing rate with the target neuron [9] , [10] . However, individual neurons recorded from the same electrode can be separately controlled in SNOC [2] , [3] , [9] , [11] . It is difficult to determine the spatial and temporal modulation in cortical activity in fine-scale (<500 μm) microcircuits using electrical recordings. Two-photon calcium imaging of cortical neurons has been used to identify multineuronal activity within a motor cortical microcircuit in rodents [12] , [13] , [14] , [15] , [16] . In contrast to SNOC in the primate, SNOC in the rodent [11] , [17] has not been performed with identification of the relations of individual neurons to physical movement. Here, we pre trained mice to perform a lever-pull movement using the right forelimb to obtain water. Then, we conducted two-photon calcium imaging of multiple neurons in layer 2/3 (L2/3) motor forelimb areas and determined whether individual neurons were related to lever-pull movement or not. Immediately after that, we conditioned the mice by reinforcing the calcium transients of a single target neuron, but not the lever-pull movement, with water delivery (SNOC by two-photon calcium imaging; 2pSNOC). We found that when the target neuron was not related to the lever-pull movement, the activity of the target neuron rapidly increased during 15 min of 2pSNOC. This increase was not accompanied by an increase in the frequency of lever-pull movements. During 2pSNOC, a subset of non-target neurons that showed high activity synchronous with reward delivery increased their activity, whereas a subset that showed high activity 2–4 s after reward delivery decreased their activity. This upward and downward modulation was recreated by repetitive channelrhodopsin-2 (ChR2) photostimulation [18] of neurons 250 ms before and 2.5 s after the reward delivery, respectively. The results indicate that reward-timing-dependent bidirectional modulation is a fundamental process in L2/3 microcircuit reorganization during fast adaptation to novel environments. Physical and neuronal operant conditioning To introduce physical operant conditioning before 2pSNOC, head-restrained mice were trained to perform a self-initiated lever-pull task using the right forelimb [13] , [16] , [19] . A 4-μl water drop was provided as a reward when the lever was pulled for 0.4 s after being left in the wait position for >3 s ( Fig. 1a ) [13] . An adeno-associated virus (AAV) encoding a calcium indicator, GCaMP7 [20] , was injected into the left motor forelimb areas [13] , [21] , [22] 1–2 weeks before the start of the lever-pull task-training sessions. After 5–14 lever-pull task-training sessions (one session per day), two-photon calcium imaging of L2/3 motor cortical neurons was performed while mice performed 2pSNOC. A total of 24 2pSNOC sessions were recorded in seven mice (one to eight sessions per mouse). Each 2pSNOC session consisted of three periods ( Fig. 1b ): a pre-conditioning period (10 min), a conditioning period (15 min) and a post-conditioning period (10 min). 2pSNOC was performed during the conditioning period. 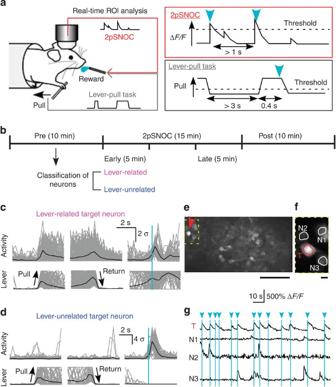Figure 1: Single-neuron operant conditioning. (a) A head-restrained mouse was provided with a water reward every time a calcium transient in the target neuron exceeded a threshold (2pSNOC task, top right; red) or every time the mouse successfully pulled a lever (lever-pull task, bottom right; grey). In the 2pSNOC task, one computer controlled two-photon imaging and another was used to analyze fluorescence intensity of a region of interest (ROI) containing a target neuron and control water delivery. Cyan arrowheads denote reward delivery. (b) The timeline for a 2pSNOC session showing the three imaging periods. (c,d) Activity of a representative lever-related target neuron (c) and a representative lever-unrelated target neuron (d) aligned to lever-pull onset (left), lever-return end (middle) and reward delivery (vertical cyan bar, right) during all three imaging periods. The lever trajectory is shown below the neuron activity. The thick black traces denote the mean of all traces. (e) A time-averaged image of a representative L2/3 field during the 2pSNOC task. Red arrowhead indicates the target neuron. Scale bar, 100 μm. (f) Expanded image of the rectangle in panele. ROIs for the target neuron (T) and three neighboring neurons (N1, N2 and N3) are overlaid. Scale bar, 10 μm. (g) Relative change in fluorescence (ΔF/F) of the target neuron and the three neighboring neurons shown in panelfduring the 2pSNOC task. Vertical cyan bars denote reward delivery. Figure 1: Single-neuron operant conditioning. ( a ) A head-restrained mouse was provided with a water reward every time a calcium transient in the target neuron exceeded a threshold (2pSNOC task, top right; red) or every time the mouse successfully pulled a lever (lever-pull task, bottom right; grey). In the 2pSNOC task, one computer controlled two-photon imaging and another was used to analyze fluorescence intensity of a region of interest (ROI) containing a target neuron and control water delivery. Cyan arrowheads denote reward delivery. ( b ) The timeline for a 2pSNOC session showing the three imaging periods. ( c , d ) Activity of a representative lever-related target neuron ( c ) and a representative lever-unrelated target neuron ( d ) aligned to lever-pull onset (left), lever-return end (middle) and reward delivery (vertical cyan bar, right) during all three imaging periods. The lever trajectory is shown below the neuron activity. The thick black traces denote the mean of all traces. ( e ) A time-averaged image of a representative L2/3 field during the 2pSNOC task. Red arrowhead indicates the target neuron. Scale bar, 100 μm. ( f ) Expanded image of the rectangle in panel e . ROIs for the target neuron (T) and three neighboring neurons (N1, N2 and N3) are overlaid. Scale bar, 10 μm. ( g ) Relative change in fluorescence (Δ F / F ) of the target neuron and the three neighboring neurons shown in panel f during the 2pSNOC task. Vertical cyan bars denote reward delivery. Full size image The pre-conditioning period was used to classify the imaged neurons according to their association with the pre-trained lever-pull movement and to select a conditioned neuron (target neuron). Mice could freely pull the lever, but the reward corresponding to a successful lever-pull for the lever-pull task (>0.4 s pull with >3 s wait) was omitted to avoid satiation. A successful lever-pull that did not directly induce the reward was defined as a virtual hit. Virtual hits occurred at a frequency of 1.9±0.1 min −1 during the pre-conditioning period ( n =24 sessions from seven mice), possibly because of partial habituation and/or expectation of reward. Many neurons exhibited large calcium transients related to the lever-pull movement, similar to our previous report [13] . According to the value of normalized non-negative deconvolution [23] of each relative fluorescent change (Δ F / F ) trace (‘activity’; see Methods), active neurons during the pre-conditioning period were reconstructed (35.0±16.4 neurons, n =24 sessions from seven mice) and classified into two groups: neurons with high activity during lever-related periods (from 1 s before the onset of lever-pull to 3 s after the end of lever-pull; ‘lever-related neurons’) ( Fig. 1c ), and other neurons (‘lever-unrelated neurons’) ( Fig. 1d ). Most reconstructed neurons were assumed to be excitatory neurons because GCaMP expression was under the control of synapsin I promoter, which considerably limits the expression to excitatory neurons [16] , [24] . One neuron was targeted in the conditioning period. This target neuron was a lever-related neuron in 13 sessions and a lever-unrelated neuron in 11 sessions. During the conditioning period, the mouse performed a 2pSNOC task. During the 2pSNOC task, two 4-μl water drops were delivered to the mouse immediately after the Δ F / F of a single target neuron increased above a threshold ( Fig. 1a,e–g ). A water reward was delivered after a calcium transient in the target neuron, irrespective of whether the target neuron was lever-related or lever-unrelated ( Fig. 1c,d ). Calcium transients in nearby neurons did not trigger reward delivery ( Fig. 1f,g ). Ninety-eight percent of the water rewards were given immediately after the calcium transient in the target neuron exceeded the threshold (1,000 successful rewards from 1,020 total rewards in 24 sessions from seven mice). The remaining 2% of rewards were delivered when Δ F / F exceeded the threshold without an obvious calcium transient. The latency from the calcium transient in the target neuron to the corresponding reward delivery was 212±122 ms ( n =1,000 successful rewards), which, when compared with values reported in a previous study, was sufficiently fast for operant conditioning [25] . Rapid activity changes in target neurons during SNOC First, we examined whether reward delivery corresponding to calcium transients in lever-related and lever-unrelated target neurons resulted in rapid changes in the activity of the target neuron during the 15 min conditioning period. For lever-unrelated target neurons, activity increased by ~50%, whereas, for lever-related target neurons, activity did not change ( Fig. 2a,b ). Activity gain was defined as the ratio of the mean activity in the last 5 min of the conditioning period (late conditioning period) to the mean activity in the first 5 min of the conditioning period (early conditioning period) minus 1. When activity gain was averaged across sessions and/or neurons, the logarithmic mean of the ratio was used ( Fig. 2c ). For lever-unrelated target neurons, the activity gain was substantially above zero ( Fig. 2d and Table 1 ). For lever-related target neurons, activity gain was not different from zero ( Fig. 2d and Table 1 ). This pattern remained even after exclusion of the mouse in which eight sessions were performed, with a mean activity gain of 55.3% and −0.73% in lever-unrelated and lever-related target neurons, respectively. 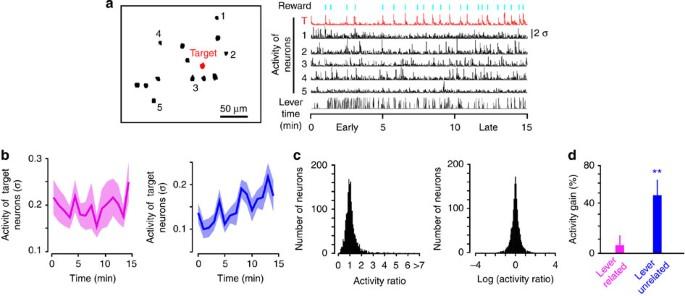Figure 2: Neuronal activity during optical single-neuron operant conditioning. (a) Left, an example of the imaged field. T (red) indicates the lever-unrelated target neuron. Black indicates the non-target neurons that were simultaneously monitored. Right, non-negatively deconvoluted ΔF/F(activity) of the target neuron and five representative non-target neurons during the 15-min conditioning period. The activity isZscored for each neuron. Vertical cyan bars denote reward delivery. (b) Time course of the activity of lever-related (left;n=13) and lever-unrelated (right;n=11) target neurons during the conditioning period. The activity isZscored for each neuron. Thick lines and shading indicate the mean±s.e.m. (c) Left, a histogram of the activity ratio from all reconstructed neurons (n=840 from 24 sessions from seven mice), where the activity ratio for each neuron was calculated as the mean activity in the first 5 min of the conditioning period divided by that in the last 5 min of the conditioning period or the mean activity in the last 5 min divided by that in the first 5 min. When all activity ratios were summed and then divided by the number of neurons, the mean value was 1.13; significantly larger than one (P<10−8,t-test). Thus, if the linear sum of the activity ratio divided by the neuron number is used as the mean, the mean is positive. Right, a histogram of the log-scaled activity ratio. The mean was zero by definition and the s.d. was 0.46. Thus, the logarithmic mean of the ratio of the mean activity in the last 5 min divided by that in the early 5 min was used for averaging. (d) Activity gain of lever-related and lever-unrelated target neurons (lever-related,P=0.43,n=13; lever-unrelated, **P=0.0039,n=11; one-samplet-test compared with zero). Figure 2: Neuronal activity during optical single-neuron operant conditioning. ( a ) Left, an example of the imaged field. T (red) indicates the lever-unrelated target neuron. Black indicates the non-target neurons that were simultaneously monitored. Right, non-negatively deconvoluted Δ F / F (activity) of the target neuron and five representative non-target neurons during the 15-min conditioning period. The activity is Z scored for each neuron. Vertical cyan bars denote reward delivery. ( b ) Time course of the activity of lever-related (left; n =13) and lever-unrelated (right; n =11) target neurons during the conditioning period. The activity is Z scored for each neuron. Thick lines and shading indicate the mean±s.e.m. ( c ) Left, a histogram of the activity ratio from all reconstructed neurons ( n =840 from 24 sessions from seven mice), where the activity ratio for each neuron was calculated as the mean activity in the first 5 min of the conditioning period divided by that in the last 5 min of the conditioning period or the mean activity in the last 5 min divided by that in the first 5 min. When all activity ratios were summed and then divided by the number of neurons, the mean value was 1.13; significantly larger than one ( P <10 −8 , t -test). Thus, if the linear sum of the activity ratio divided by the neuron number is used as the mean, the mean is positive. Right, a histogram of the log-scaled activity ratio. The mean was zero by definition and the s.d. was 0.46. Thus, the logarithmic mean of the ratio of the mean activity in the last 5 min divided by that in the early 5 min was used for averaging. ( d ) Activity gain of lever-related and lever-unrelated target neurons (lever-related, P =0.43, n =13; lever-unrelated, ** P =0.0039, n =11; one-sample t -test compared with zero). Full size image Table 1 The mean activity gain of each type of target neuron. Full size table Next, we determined whether operant conditioning of the target neuron increased the frequency of reward delivery induced by calcium transients above the threshold. As expected, the reward frequency increased by ~50% when lever-unrelated neurons were targeted, and did not change when lever-related neurons were targeted ( Fig. 3a ). Similar to activity gain, reward gain was defined as the ratio of the reward frequency in the late conditioning period to the reward frequency in the early conditioning period minus 1, and the logarithmic mean of the ratio was used for averaging ( Fig. 3b ). The reward gain was substantially above zero when lever-unrelated neurons were targeted, and was not different from zero when lever-related neurons were targeted ( Fig. 3c ). The activity gain and the reward gain were correlated in both types of target neurons ( Fig. 3d ). When lever-unrelated neurons were targeted, activity gain was positive in all 11 sessions (from five mice) and reward gain was positive in 8 of the 11 sessions; therefore, the mouse steadily increased the target neuron activity and reward frequency. 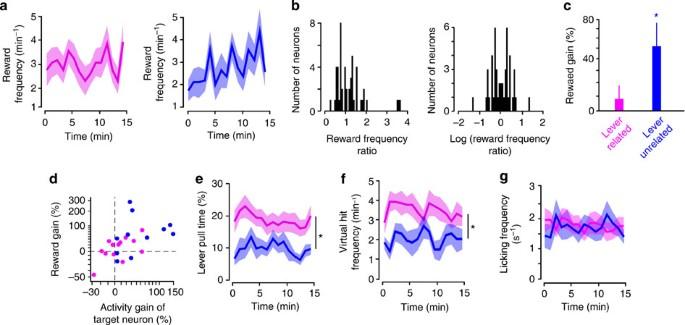Figure 3: Reward frequency and behaviours during optical single-neuron operant conditioning. (a) Time course of the reward frequency when lever-related (left;n=13) and lever-unrelated (right;n=11) neurons were targeted. Thick lines and shading indicate the mean±s.e.m. (b) Left, a histogram of the reward frequency ratio from all sessions (n=24 sessions from seven mice), where the reward frequency ratio was calculated as the mean reward frequency in the first 5 min divided by that in the last 5 min or the mean reward frequency in the last 5 min divided by that in the first 5 min. Right, a histogram of the log-scaled reward frequency ratio. (c) Reward gain when lever-related and lever-unrelated neurons were targeted (lever-related,P=0.37,n=13; lever-unrelated, *P=0.020,n=11; one-samplet-test compared with zero). (d) The reward gain as a function of the activity gain of the target neurons. Each circle indicates a different session. Magenta, lever-related target neurons. Blue, lever-unrelated target neurons. (Pearson’s correlation coefficient=0.54,P=0.0065,n=24 sessions). (e) Time course of the percentage of time spent pulling the lever when lever-related (magenta,n=13) and lever-unrelated (blue,n=11) neurons were targeted. Thick lines and shading indicate the mean±s.e.m. *P=0.011; Wilcoxon rank sum test. (f) Time course of the frequency of virtual hits when lever-related (magentan=13) and lever-unrelated (bluen=11) neurons were targeted. Thick lines and shading indicate the mean±s.e.m. *P=0.013; Wilcoxon rank sum test. (g) Time course of the frequency of licking when lever-related (magenta,n=13) and lever-unrelated (blue,n=11) neurons were targeted. Thick lines and shading indicate the mean±s.e.m. Figure 3: Reward frequency and behaviours during optical single-neuron operant conditioning. ( a ) Time course of the reward frequency when lever-related (left; n =13) and lever-unrelated (right; n =11) neurons were targeted. Thick lines and shading indicate the mean±s.e.m. ( b ) Left, a histogram of the reward frequency ratio from all sessions ( n =24 sessions from seven mice), where the reward frequency ratio was calculated as the mean reward frequency in the first 5 min divided by that in the last 5 min or the mean reward frequency in the last 5 min divided by that in the first 5 min. Right, a histogram of the log-scaled reward frequency ratio. ( c ) Reward gain when lever-related and lever-unrelated neurons were targeted (lever-related, P =0.37, n =13; lever-unrelated, * P =0.020, n =11; one-sample t -test compared with zero). ( d ) The reward gain as a function of the activity gain of the target neurons. Each circle indicates a different session. Magenta, lever-related target neurons. Blue, lever-unrelated target neurons. (Pearson’s correlation coefficient=0.54, P =0.0065, n =24 sessions). ( e ) Time course of the percentage of time spent pulling the lever when lever-related (magenta, n =13) and lever-unrelated (blue, n =11) neurons were targeted. Thick lines and shading indicate the mean±s.e.m. * P =0.011; Wilcoxon rank sum test. ( f ) Time course of the frequency of virtual hits when lever-related (magenta n =13) and lever-unrelated (blue n =11) neurons were targeted. Thick lines and shading indicate the mean±s.e.m. * P =0.013; Wilcoxon rank sum test. ( g ) Time course of the frequency of licking when lever-related (magenta, n =13) and lever-unrelated (blue, n =11) neurons were targeted. Thick lines and shading indicate the mean±s.e.m. Full size image Next, we examined the specificity of the target neuron. The mean activity gain of the non-target neurons was slightly larger than zero when a lever-unrelated neuron was targeted and slightly smaller than zero when a lever-related neuron was targeted ( Table 2 ). To examine whether the relative change in activity of the target neuron from the early to the late conditioning period exceeded that in the non-target neurons, we ranked the activity of the target neuron among all reconstructed neurons, including target and non-target neurons. The rank was normalized between 1 (top) and 100 (bottom) in the early and late conditioning periods during each session. When a lever-unrelated neuron was targeted, the normalized rank of the target neuron significantly rose from the early to the late conditioning period (change in normalized rank, 18.0±6.4; P =0.0078, Wilcoxon signed-rank test; n =11). When a lever-related neuron was targeted, the normalized rank of the target neuron was similar in the early and late conditioning periods (change in normalized rank, 4.5±4.1; P =0.56, Wilcoxon signed-rank test; n =13). Thus, both of the activity and rank of the target neuron significantly increased from the early to the late conditioning period when a lever-unrelated neuron was targeted. These results indicate that the rapid operant conditioning of single lever-unrelated neurons was successful even though the activity of non-target neurons slightly changed. By contrast, the rapid operant conditioning of single lever-related neurons was not successful. Table 2 The mean activity gain of each type of non-target neuron. Full size table In lever-related neurons, calcium transients would coincide with a lever-pull. In the 2pSNOC, mice were rewarded for calcium transients in the target neuron. Therefore, when lever-related neurons were targeted, pulling the lever would result in the delivery of a reward, meaning that the mice did not have to change the strategy that they adopted in the lever-pull task to get rewards during the conditioning period. In support of this, the amount of time spent pulling the lever and the frequency of virtual hits in the conditioning period were approximately twofold larger when lever-related neurons were targeted than when lever-unrelated neurons were targeted ( Fig. 3e,f ), although licking frequency was not different ( Fig. 3g ). Irrespective of the target neuron type, lever-pull behaviours did not change from the early to the late conditioning period. These results suggest that, when lever-related neurons were targeted, the mouse performed goal-directed lever-pull movements from the onset of the conditioning period without recognition of SNOC. This may explain why the activity gain for lever-related target neurons was not significantly positive. In the following analyses of the microcircuit reorganization during 2pSNOC, only data from sessions with a lever-unrelated target neuron were used (11 sessions from five mice; n =381 non-target neurons). Reward-timing-dependent bidirectional modulation Next, we examined whether non-target neurons associated with the target neuron changed their activity more markedly than other non-target neurons. The activity gain was similar for lever-related non-target neurons and lever-unrelated non-target neurons ( Fig. 4a and Table 2 ). The activity gain of non-target neurons was not associated with the distance to the target neuron ( Fig. 4b ). By contrast, the activity gain of non-target neurons was weakly related to the pairwise correlation with the target neuron during the conditioning period (excluding the reward-related periods from 0 to 5 s after each reward delivery; spontaneous pairwise correlation) ( Fig. 4c ). This indicates that non-target neurons whose activity was temporally, but not spatially, associated with the target neuron increased their activity, although the strength of the spontaneous pairwise correlation was negatively associated with the cellular distance ( Fig. 4d ), as previously reported in the mouse motor cortex [12] , [13] , [15] . 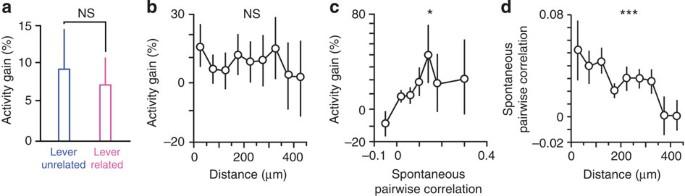Figure 4: Modulation of non-target neurons. (a) Activity gain of lever-unrelated (blue,n=226) and lever-related (magenta,n=155) non-target neurons. NS indicates no significant difference (P=0.74; two-samplet-test). (b) Activity gain of non-target neurons as a function of the distance from the target neuron (Spearman’s correlation coefficient (r)=−0.0077,P=0.88,n=381). (c) Activity gain of non-target neurons as a function of the strength of the spontaneous pairwise correlation with the target neuron during the conditioning period (r=0.10, *P=0.043,n=381). (d) Strength of the spontaneous pairwise correlation between each non-target neuron and the target neuron during the conditioning period as a function of distance between the two neurons (r=–0.22, ***P=1.8 × 10−5,n=381). Figure 4: Modulation of non-target neurons. ( a ) Activity gain of lever-unrelated (blue, n =226) and lever-related (magenta, n =155) non-target neurons. NS indicates no significant difference ( P =0.74; two-sample t -test). ( b ) Activity gain of non-target neurons as a function of the distance from the target neuron (Spearman’s correlation coefficient ( r )=−0.0077, P =0.88, n= 381). ( c ) Activity gain of non-target neurons as a function of the strength of the spontaneous pairwise correlation with the target neuron during the conditioning period ( r =0.10, * P =0.043, n= 381). ( d ) Strength of the spontaneous pairwise correlation between each non-target neuron and the target neuron during the conditioning period as a function of distance between the two neurons ( r =–0.22, *** P =1.8 × 10 −5 , n =381). Full size image Although the change in the activity of non-target neurons was weakly associated with the correlation with the target neuron, non-target neurons should have been affected by the water delivery because it was the reinforcer. Therefore, we next investigated whether the activity gain was affected by the activity timing of the non-target neurons relative to the reward delivery ( Fig. 5a ). For each non-target neuron, the ratio of the sum of the activity in a 0.33-s time bin t s after reward delivery during the first 10 min of the conditioning period to the sum of the remaining activity in the same bin during the first 10 min of the conditioning period was defined as the reward synchronization index ( t ) (RSI( t ); see Methods for details). For each time bin, activity gain was averaged across the non-target neurons with RSI values in the top 5% ( Fig. 5b ). The activity gain of non-target neurons with RSI in the top 5% was significantly larger than zero when t ranged from −0.33 s to 0.33 s, and significantly smaller than zero when t was 2.3, 3 and 4 s ( Fig. 5c ). We refer to this phenomenon as reward-timing-dependent bidirectional modulation (RTBM), and refer to neurons that had at least one RSI (−0.33 s to 0.33 s) in the top 5% as reward-synchronous active (SR) neurons ( n =34) and neurons that had at least one RSI (2–4 s) in the top 5% as after-reward active (AR) neurons ( n =39). Neurons that met both criteria were categorized according to the time bin with the highest RSI. The activity gain of SR and AR neurons was substantially positive and negative, respectively ( Fig. 5d ). RTBM was also detected when RSI values that determined SR and AR neurons ranged from the top 2% to the top 10% ( Fig. 5e ). In addition, RTBM was observed when neurons with RSI in the top 20% for each time bin in each session were selected; the activity gain of neurons with RSI (0 s) in the top 20% (SR 20% neurons) averaged across-sessions was substantially higher than zero and that of neurons with RSI (2.3 s) in the top 20% (AR 20% neurons) averaged across-sessions ( Fig. 5f ). In 9 of 10 sessions with >2 SR 20% neurons and >2 AR 20% neurons (five, two, one, and one out of five, two, two and one sessions from four mice, respectively), the mean activity gain of SR 20% neurons was higher than that of AR 20% neurons; thus, the timing of neuronal activity relative to the reward was a critical factor in the modulation of the two groups of non-target neurons. 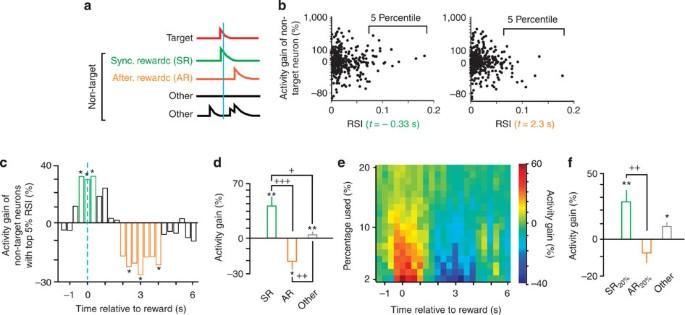Figure 5: Reward-timing-dependent bidirectional modulation. (a) Activity of target neurons (red), non-target neurons with high activity around reward delivery (green) or after reward delivery (orange) and other non-target neurons (black). (b) Activity gain of non-target neurons as a function of the reward synchronization index (RSI) at 0.33 s before (left) and 2.3 s after (right) reward delivery. (c) Mean activity gain of non-target neurons with RSI in the top 5% as a function of the RSI time bin. Vertical cyan dashed line denotes reward timing. Asterisks indicateP<0.05 (one-samplet-test compared with zero). Green and orange bars indicate the time bins used to determine reward-synchronous active (SR) and after-reward active (AR) neurons, respectively. (d) Mean activity gain of SR, AR and other non-target neurons. SR,P=0.0017,n=34; AR,P=0.010,n=39; other non-target,P=0.0014,n=308; one-samplet-test compared with zero. *P<0.05, **P<0.01. One-way ANOVA indicated a significant difference across neuron types (P=6.7 × 10−5).+P=0.049,++P=0.0014,+++P=4.1 × 10−5;post-hocHSD test. (e) Mean activity gain of non-target neurons with the top 2–20% RSI from the pooled data as a function of the RSI time bin relative to reward delivery. The activity gain is pseudo-colour coded. (f) Mean activity gains of SR20%, AR20%and other non-target neurons, where non-target neurons with the top 20% RSI (t=0 s andt=2.3 s) in each session were defined as SR20%neurons (green) and AR20%neurons (orange), respectively (SR20%, **P=0.0026,n=74; AR20%,P=0.19,n=74; the other non-target neurons, *P=0.021,n=233, one-samplet-test compared with zero). The activity gain of SR20%neurons was significantly larger than that of AR20%neurons (P=0.0022, one-way ANOVA,++P=0.0013,post hocHSD test). Figure 5: Reward-timing-dependent bidirectional modulation. ( a ) Activity of target neurons (red), non-target neurons with high activity around reward delivery (green) or after reward delivery (orange) and other non-target neurons (black). ( b ) Activity gain of non-target neurons as a function of the reward synchronization index (RSI) at 0.33 s before (left) and 2.3 s after (right) reward delivery. ( c ) Mean activity gain of non-target neurons with RSI in the top 5% as a function of the RSI time bin. Vertical cyan dashed line denotes reward timing. Asterisks indicate P <0.05 (one-sample t -test compared with zero). Green and orange bars indicate the time bins used to determine reward-synchronous active (SR) and after-reward active (AR) neurons, respectively. ( d ) Mean activity gain of SR, AR and other non-target neurons. SR, P =0.0017, n =34; AR, P =0.010, n =39; other non-target, P =0.0014, n =308; one-sample t -test compared with zero. * P <0.05, ** P <0.01. One-way ANOVA indicated a significant difference across neuron types ( P =6.7 × 10 −5 ). + P =0.049, ++ P =0.0014, +++ P =4.1 × 10 −5 ; post-hoc HSD test. ( e ) Mean activity gain of non-target neurons with the top 2–20% RSI from the pooled data as a function of the RSI time bin relative to reward delivery. The activity gain is pseudo-colour coded. ( f ) Mean activity gains of SR 20% , AR 20% and other non-target neurons, where non-target neurons with the top 20% RSI ( t =0 s and t =2.3 s) in each session were defined as SR 20% neurons (green) and AR 20% neurons (orange), respectively (SR 20% , ** P =0.0026, n =74; AR 20% , P =0.19, n =74; the other non-target neurons, * P =0.021, n =233, one-sample t -test compared with zero). The activity gain of SR 20% neurons was significantly larger than that of AR 20% neurons ( P =0.0022, one-way ANOVA, ++ P =0.0013, post hoc HSD test). Full size image We next examined the association between SR and AR neurons and the target neuron. The percentage of lever-related and lever-unrelated neurons was similar between SR and AR neurons ( Fig. 6a ) and the distance of SR and AR neurons from the target neuron was similar to the distance of other neurons from the target neuron ( Fig. 6b ). The pairwise correlation with the target neuron was higher for SR neurons than for AR neurons and other neurons during both the conditioning and pre-conditioning periods, that is, without water delivery ( Fig. 6c ). This is consistent with the result shown in Fig. 4c and indicates that SR neurons were frequently active together with the target neuron because the reward delivery was induced by a calcium transient in the target neuron beyond the threshold with only ~200 ms delay. Thus, SR neurons, which were highly correlated with the target neuron, exhibited an increase in activity irrespective of whether the activity was lever-related, or the distance from the target neuron. By contrast, AR neurons did not appear different from other non-target neurons in terms of their associations with the target neuron. 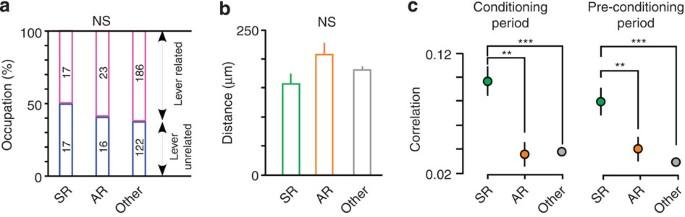Figure 6: Characteristics of neurons with reward-timing-dependent bidirectional modulation. (a) Percentage of lever-related (magenta) and lever-unrelated (blue) neurons. The number inside each bar denotes the total number of neurons. SR versus AR,P=0.44; AR versus other,P=0.85; other versus SR,P=0.23;χ2-test. (b) Distance of SR, AR and other non-target neurons from the target neuron. SR versus AR,P=0.084; AR versus other,P=0.22; other versus SR,P=0.26; Wilcoxon rank sum test. (c) The spontaneous pairwise correlation of SR, AR and other non-target neurons with the target neuron during the conditioning period (left) and pre-conditioning period (right). Left: SR versus AR, **P<2.3 × 10−5; AR versus other,P=0.31; other versus SR, ***P=4.8 × 10−7; Wilcoxon rank sum test. Right: SR versus AR, **P=0.008; AR versus other,P=0.53; other versus SR, ***P=1.9 × 10−5; Wilcoxon rank sum test. Figure 6: Characteristics of neurons with reward-timing-dependent bidirectional modulation. ( a ) Percentage of lever-related (magenta) and lever-unrelated (blue) neurons. The number inside each bar denotes the total number of neurons. SR versus AR, P =0.44; AR versus other, P =0.85; other versus SR, P =0.23; χ 2 -test. ( b ) Distance of SR, AR and other non-target neurons from the target neuron. SR versus AR, P =0.084; AR versus other, P =0.22; other versus SR, P =0.26; Wilcoxon rank sum test. ( c ) The spontaneous pairwise correlation of SR, AR and other non-target neurons with the target neuron during the conditioning period (left) and pre-conditioning period (right). Left: SR versus AR, ** P <2.3 × 10 −5 ; AR versus other, P =0.31; other versus SR, *** P =4.8 × 10 −7 ; Wilcoxon rank sum test. Right: SR versus AR, ** P =0.008; AR versus other, P =0.53; other versus SR, *** P =1.9 × 10 −5 ; Wilcoxon rank sum test. Full size image Neither SR nor AR neurons were specifically related to licking because licking frequency around the reward (–1 to 1 s) or after the reward (2 to 4 s) did not change from the early to the late conditioning period ( Fig. 7a ). Likewise, neither SR nor AR neurons were specifically related to lever-pull in response to the reward delivery because the percentage of lever-pull time and the probability of lever pulling around the reward (–1 to 1 s) and after the reward (2 to 4 s) did not change from the early to the late conditioning period ( Fig. 7b,c ). Therefore, the activity changes in AR or SR neurons cannot be explained by a gradual loss of the pre-trained memory for the mouse to pull the lever 3 s after the reward delivery. 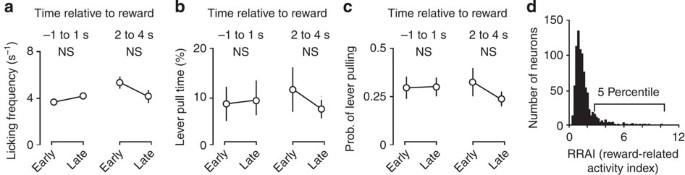Figure 7: Behaviours around and after reward delivery and the distribution of reward-related activity index. (a) Licking frequency around the time of reward delivery (–1 to 1 s) and 2 to 4 s after reward delivery in the early and late conditioning periods. −1 to 1 s,P=0.12,n=11; 2 to 4 s,P=0.15,n=11; Wilcoxon signed-rank test. (b) Lever-pull time around the time of reward delivery (–1 to 1 s) and 2 to 4 s after reward delivery in the early and late conditioning periods. Lever-pull time did not significantly change from the early to the late conditioning period (–1 to 1 s,P=0.52,n=11; 2 to 4 s,P=0.52,n=11; Wilcoxon signed-rank test). (c) The probability of lever pulling around the time of reward delivery (–1 to 1 s) and 2 to 4 s after reward delivery in the early and late conditioning periods. The probability of lever pulling did not significantly change from the early to the late period (–1 to 1 s,P=0.73,n=11; 2 to 4 s,P=0.65,n=11; Wilcoxon signed-rank test). (d) The histogram for reward-related activity index (RRAI) in non-target neurons in sessions with a lever-unrelated target neuron. Note that the distribution was strongly skewed. The non-target neurons with the top 5% RRAI were defined as reward-related neurons. Figure 7: Behaviours around and after reward delivery and the distribution of reward-related activity index. ( a ) Licking frequency around the time of reward delivery (–1 to 1 s) and 2 to 4 s after reward delivery in the early and late conditioning periods. −1 to 1 s, P =0.12, n =11; 2 to 4 s, P =0.15, n =11; Wilcoxon signed-rank test. ( b ) Lever-pull time around the time of reward delivery (–1 to 1 s) and 2 to 4 s after reward delivery in the early and late conditioning periods. Lever-pull time did not significantly change from the early to the late conditioning period (–1 to 1 s, P =0.52, n =11; 2 to 4 s, P =0.52, n =11; Wilcoxon signed-rank test). ( c ) The probability of lever pulling around the time of reward delivery (–1 to 1 s) and 2 to 4 s after reward delivery in the early and late conditioning periods. The probability of lever pulling did not significantly change from the early to the late period (–1 to 1 s, P =0.73, n =11; 2 to 4 s, P =0.65, n =11; Wilcoxon signed-rank test). ( d ) The histogram for reward-related activity index (RRAI) in non-target neurons in sessions with a lever-unrelated target neuron. Note that the distribution was strongly skewed. The non-target neurons with the top 5% RRAI were defined as reward-related neurons. Full size image We also estimated whether reward-related activity accounted for the activity gain of SR and AR neurons. The reward-related activity index (RRAI) was defined as the mean activity during the reward-related period divided by the mean activity during the non-reward-related periods of the conditioning period. Reward-related neurons were defined as the neurons with the top 5% of RRAI values because these neurons contributed to the skewed distribution of RRAI ( Fig. 7d ). As expected, the reward-related neurons tended to have positive activity gain (27.0%, P =0.14, n =19, one-sample t -test). The proportion of SR and AR neurons that were reward related was similar (14.8% for SR neurons, 23.1% for AR neurons; P =0.36, χ 2 -test). The proportion of lever-related and lever-unrelated neurons that were reward related was also similar (5.8% for lever-related neurons, 3.9% for lever-unrelated neurons; P =0.41, χ 2 -test). Thus, it was the timing of the activity relative to the reward delivery rather than the magnitude of activity induced by reward delivery that was critically involved in the microcircuit reorganization. The inter-reward interval time was 26.8±3.7 s ( n =11 sessions), which was much longer than the interval between the reward and the AR neuron activity (~2.5 s), indicating that it was unlikely that the decrease in AR neuron activity from the early to the late conditioning period occurred because these neurons had the weakest relation to the reward of all non-target neurons. Rather, these results suggest that the activity of AR neurons decreased owing to the timing (~2.5 s) of the activity relative to reward delivery. Pairing of ChR2 photostimulation and reward recreated RTBM To validate whether the activity timing relative to the reward delivery is sufficient to induce the neuronal activity changes, we performed repetitive pairing of the activity of a random set of neurons and reward delivery with different time intervals. We expressed GCaMP6f [26] in a majority of the neurons and ChR2-mCherry [18] in a subset of neurons to be photostimulated ( Fig. 8a ; see Methods). The photostimulation was performed in mice that had not been trained to perform the lever-pull task. In each photostimulation session, 60 photostimuli were delivered during a 15 min period to induce firing in ChR2-mCherry-expressing neurons in the field of view and a reward (8 μl of water) was given 0.25 s after or 2.5 s before each photostimulation (potentiation protocol and depression protocol, respectively) ( Fig. 8b ). Photostimulation did not induce any observable movements. To prevent visual associative learning between the photostimulation and the reward, a blue-light-emitting diode was illuminated in front of both eyes every 2–3 s. Two-photon calcium imaging was conducted during the photostimulation period. For each reconstructed neuron, photostimuli-induced activity gain was quantified as the ratio of the mean Δ F / F in the last 5 min of the photostimulation period to that in the first 5 min minus 1. We identified neurons that showed significantly higher activity in response to the ChR2 photostimuli than to the light-emitting diode illuminations ( P <0.05; one-tailed two-sample t -test) and termed them photostimuli-responsive neurons ( Fig. 8c ). In the potentiation protocol, 56% of imaged neurons were photostimuli-responsive neurons (78 out of 139 neurons in four sessions from four mice), whereas, in the depression protocol, 30% of imaged neurons were photostimuli-responsive neurons (40 out of 132 neurons in four sessions from four mice). Although the photostimuli-responsive neurons in these two protocols had almost identical Δ F / F at the beginning of the sessions, the photostimuli-induced activity gains of these neurons were significantly positive and negative in the potentiation and depression protocols, respectively ( Fig. 8d,e ). The activity gain of the other neurons was not significantly different from zero in either protocol (potentiation protocol, P =0.059, n =61; depression protocol, P =0.20, n =92; one-sample t -test). The different modulation of photostimuli-responsive neurons in the potentiation and depression protocols was not due to a difference in licking behaviours because the licking frequency around the reward (–1 to –1 s) and after the reward (2 to 4 s) did not change from the first 5 min to the last 5 min in either protocol ( Fig. 8f ). In addition, 60 photostimuli delivered without any water delivery did not induce substantial changes in the activity gain in the photostimuli-responsive neurons ( Fig. 8e ); thus, repetitive pairing of neuronal activity with reward delivery at different time intervals was sufficient to recreate RTBM. 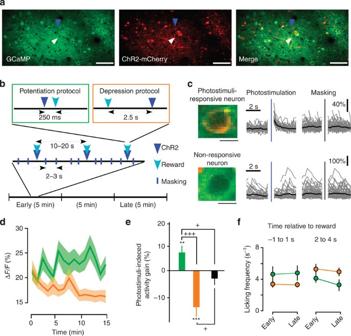Figure 8: Repetitive pairing of the reward and photostimulation altered the activity of photostimuli-responsive neurons. (a) Example images of GCaMP6f (left), ChR2-mCherry (middle) and their overlay (right) in the same field. Scale bars, 50 μm. Blue arrowheads indicate a GCaMP6f-positive and mCherry-positive neuron. White arrowheads indicate a GCaMP6f-positive and mCherry-negative neuron. (b) Protocols for delivering ChR2 stimuli. Blue and cyan arrowheads indicate ChR2 stimuli and reward deliveries, respectively. For masking (blue bars), a blue light was illuminated in front of the eyes every 2–3 s. (c) Left: Expanded images of the photostimuli-responsive neuron indicated by blue arrowheads in panela(top) and the photostimuli-non-responsive neuron indicated by white arrowheads in panela(bottom). Scale bars, 5 μm. Right: ΔF/Ftraces of these neurons aligned with ChR2 photostimulation (blue line; middle) and light masking (black line; right). The thick black traces denote the mean of all traces. Broken points in the grey traces indicate the time of unaligned masking. (d) Time course of the mean ΔF/Fof photostimuli-responsive neurons in the potentiation (green,n=78 neurons) and depression (orange,n=40 neurons) protocols. Thick lines and shading indicate the mean±s.e.m. (e) Photostimuli-induced activity gain of the photostimuli-responsive neurons in the potentiation protocol (left, green;n=78 in four sessions from four mice) and depression protocol (middle, orange;n=40 in four sessions from four mice) and 60 photostimuli without reward (right, black;n=77 in four sessions from three mice). Potentiation,**P=0.0081; depression, ***P=0.00040; no-reward,P=0.26; one-samplet-test compared with zero. One-way analysis of variance indicated a significant difference across protocols (P=1.8 × 10−5). Crosses indicate the results ofpost-hocpairwise comparisons: potentiation versus depression,+++P=6.1 × 10−6; depression versus no-reward,+P=0.032; no-reward versus potentiation,+P=0.019; HSD test. (f) Licking frequency around the time of reward delivery (–1 to 1 s) and 2 to 4 s after reward delivery in the early and late conditioning periods. Green, potentiation protocol (n=4). Orange, depression protocol (n=4). Figure 8: Repetitive pairing of the reward and photostimulation altered the activity of photostimuli-responsive neurons. ( a ) Example images of GCaMP6f (left), ChR2-mCherry (middle) and their overlay (right) in the same field. Scale bars, 50 μm. Blue arrowheads indicate a GCaMP6f-positive and mCherry-positive neuron. White arrowheads indicate a GCaMP6f-positive and mCherry-negative neuron. ( b ) Protocols for delivering ChR2 stimuli. Blue and cyan arrowheads indicate ChR2 stimuli and reward deliveries, respectively. For masking (blue bars), a blue light was illuminated in front of the eyes every 2–3 s. ( c ) Left: Expanded images of the photostimuli-responsive neuron indicated by blue arrowheads in panel a (top) and the photostimuli-non-responsive neuron indicated by white arrowheads in panel a (bottom). Scale bars, 5 μm. Right: Δ F / F traces of these neurons aligned with ChR2 photostimulation (blue line; middle) and light masking (black line; right). The thick black traces denote the mean of all traces. Broken points in the grey traces indicate the time of unaligned masking. ( d ) Time course of the mean Δ F / F of photostimuli-responsive neurons in the potentiation (green, n =78 neurons) and depression (orange, n =40 neurons) protocols. Thick lines and shading indicate the mean±s.e.m. ( e ) Photostimuli-induced activity gain of the photostimuli-responsive neurons in the potentiation protocol (left, green; n =78 in four sessions from four mice) and depression protocol (middle, orange; n =40 in four sessions from four mice) and 60 photostimuli without reward (right, black; n =77 in four sessions from three mice). Potentiation, **P =0.0081; depression, *** P =0.00040; no-reward, P =0.26; one-sample t -test compared with zero. One-way analysis of variance indicated a significant difference across protocols ( P =1.8 × 10 −5 ). Crosses indicate the results of post-hoc pairwise comparisons: potentiation versus depression, +++ P =6.1 × 10 −6 ; depression versus no-reward, + P =0.032; no-reward versus potentiation, + P =0.019; HSD test. ( f ) Licking frequency around the time of reward delivery (–1 to 1 s) and 2 to 4 s after reward delivery in the early and late conditioning periods. Green, potentiation protocol ( n =4). Orange, depression protocol ( n =4). Full size image Here, we demonstrated rapid operant conditioning of single neurons in the rodent motor cortex by two-photon calcium imaging. The physical reward contingency task was introduced in advance, and the mice rapidly learned to increase the activity of target neurons that were not related to the pre-trained movement. The increase in the activity of these neurons was robust; the mean activity increase was ~50% of the first 5 min activity. The successful operant conditioning of lever-unrelated neurons is consistent with the fact that cortical neurons with no discernible relation to muscles can be volitionally modulated in the primate motor cortex [9] . In addition, we showed, for the first time, that the timing of neuronal activity relative to the reward is one of the critical factors for the activity change in non-target neurons in microcircuits. The modulation of non-target neurons was bidirectional and was reproduced by repetitive pairing of ChR2 photostimulation with reward. Recently, operant conditioning of two ensembles in the mouse motor cortex by two-photon calcium imaging was reported, whereby the mouse was conditioned to change the activity of the two ensembles in opposite directions [27] . The temporal dynamics of the activities in the two target ensembles were different to each other, and the conditioning depended on the correlation between them. Therefore, for each non-target neuron, the spatial and temporal associations with the target ensembles were inevitably affected not only by each target ensemble, but also by the relation between the two target ensembles. By contrast, in the present study, the target neuron was a single neuron; therefore the spatial and temporal associations with the target neuron could be unambiguously determined for each non-target neuron. Our results clearly showed that non-target neurons that exhibited high activity synchronous with reward delivery (SR neurons) were reinforced and non-target neurons whose activity followed the reward after 2–4 s (AR neurons) were repressed. The correlation between SR neurons and the target neuron was higher than that between other non-target neurons and the target neuron; however, the distance to the target neuron was similar across SR, AR and other non-target neurons. This suggests that the microcircuit has the capability to strengthen the activity of neurons that were previously included in the same ensemble without strong spatial constrains, which can explain the variety of behaviours of non-target neurons observed during SNOC in primates [2] , [3] , [9] , [10] . During fast adaptation, which requires changes in behaviours or internal models [28] , novel ensembles may be broadly generated based on the structure of pre-existing ensembles. However, our finding that lever-related and lever-unrelated non-target neurons were similarly modulated during the conditioning period suggests that pre-existing ensembles that are not relevant to a novel reward contingency do not necessarily restrict the microcircuit reorganization. We found that a subset of non-target neurons that were not correlated with the target neuron decreased their activity over the conditioning period. The changes in the activity of SR and AR neurons were not due to changes in licking or lever-pull behaviours that might be related to reward prediction. The counterbalance of microcircuit activity may play a role in maintaining a constant overall level of network activity for homeostasis [14] , [16] , [29] . Our results suggest that RTBM is possibly one of many processes that underlie rapid reorganization of the L2/3 cortical microcircuit during fast adaptation to environmental changes, which occurs during brain-machine and brain-computer interface learning, motor adaptation and skill learning. RTBM was recreated by repetitive pairing of the reward with direct stimulation of a random set of neurons in the motor cortex. Although licking behaviours did not change in either protocol, the bidirectional activity changes might be related to reward prediction and reward-absence prediction signals without appearance of any behaviours. However, the proportion of imaged neurons that were photostimuli responsive (56% and 30% in the potentiation and depression protocols, respectively) was larger than the proportion of neurons with high RRAI (~5%; Fig. 7d ). In addition, reward-modulated neurons were very rarely observed (~3%) in the rat forelimb M1 in a self-initiated lever-pull–push task [19] . It is therefore unlikely that the reward-prediction activity had a large effect on the bidirectional changes in the microcircuit. Thus, our results indicate that the motor cortex can be a causal origin of the RTBM without signals from the prefrontal and parietal cortices, which are presumably required for cognitive strategies [5] , [10] . In the auditory cortex, forward conditioning of pure tone stimulation and electrical stimulation of dopaminergic ventral tegmental neurons increased the size of the cortical area responding to the tone frequency, and backward conditioning reduced the size of the area [30] , [31] . This bidirectional remodeling may share the same underlying mechanisms as RTBM in the motor cortex, although RTBM in the motor cortex was faster. The dopaminergic projections to the motor cortex are necessary for motor learning [32] . Dopamine uptake in the prefrontal cortex takes up to 5 s [33] ; therefore, increased dopamine concentration in the motor cortex may last for the observed time interval between reward delivery and activity in AR neurons. The corticostriatal synapses also show bidirectional plasticity with dopamine release [34] , which is necessary for neuroprosthetic skill learning [35] . Dopaminergic projections to the motor cortex and striatum may cooperatively induce bidirectional modulations in L2/3 neurons. Animals All animal experiments were approved by the Institutional Animal Care and Use Committee of National Institutes of Natural Sciences, Japan. Male and female C57BL/6 mice (aged 2–4 months) were utilized for the present study. All mice were provided with food and water ad libitum and housed in a 12:12 h light–dark cycle. Mice were not used for other experiments before the study. Mice were anesthetized by intraperitoneal injection of ketamine (74 mg kg −1 ) and xylazine (10 mg kg −1 ) before an incision was made in the skin covering the neocortex. After the exposed skull was cleaned, a head plate (Tsukasa Giken, Sizuoka, Japan) was attached to the skull using dental cement (Fujiryu-to BC; GC, Tokyo, Japan, Bistite II; Tokuyama Dental, Tokyo, Japan). The surface of the intact skull was coated with dental adhesive resin cement (Super bond; Sun Medical, Shiga, Japan) to prevent drying. Mice were allowed to recover for 1 day before virus injection. The number of mice per cage was 2–5 before the head plate was attached. After that, mice were single-caged to avoid damage to the head plate and the glass window. Virus production GCaMP7 cDNA was cloned from the GCaMP7 vector [20] and inserted into pAAV (Addgene plasmid 26973; a kind gift from Dr K. Deisseroth, Stanford University) to obtain recombinant AAV type 2/1 (rAAV2/1) expressing GCaMP7. The vector plasmid (pAAV- syn -GCaMP7) contained GCaMP7 cDNA and the woodchuck hepatitis virus post-transcriptional regulatory element, which was expressed under control of the pan-neuronal human synapsin I promoter ( syn -GCaMP7). rAAV2/1- syn -GCaMP7 (AAV- syn -GCaMP7) was produced following triple-transfection of HEK293 cells with pAAV- syn -GCaMP7, an adenoviral helper plasmid pAdeno and a chimeric helper plasmid encoding AAV2 rep/AAV1 cap genes (pAAV2-1, gifted to us from Dr J. M. Wilson, University of Pennsylvania) [36] , which was mediated by calcium phosphate co-precipitation with active gassing [37] . rAAV2/1- syn -GCaMP7 was purified according to previous studies [38] , [39] . All rAAV2/9 were obtained from the University of Pennsylvania Gene Therapy Program Vector Core. Virus injection Thirty minutes before surgery, dexamethasone sodium phosphate (1.32 mg kg −1 ; to prevent cerebral edema), the antibiotics sulfadiazine (24 mg kg −1 ) and trimethoprim (4.8 mg kg −1 ) and the anti-inflammatory carprofen (6 mg kg −1 ) were administered intraperitoneally. Isoflurane (1%) inhalation was used for anesthesia throughout surgery. A 2-mm diameter circular craniotomy was made over the left rostral motor forelimb area (circle centered ~2.4 mm anterior and ~0.9 mm lateral to bregma) or the left caudal motor forelimb area (circle centered ~0.2 mm anterior and ~1.2 mm lateral to bregma). The dura mater was removed. Before virus injection, a pulled glass pipette (broken and beveled to an outer diameter of ~25–30 μm; Sutter Instruments, California, USA) and a 5 μl Hamilton syringe were back-filled with mineral oil (Nacalai Tesque, Kyoto, Japan) and front-loaded with virus solution. Either 50 nl of AAV- syn -GCaMP7 (7.1 × 10 12 vector genomes ml −1 ) or 50 nl of mixed solution containing AAV- syn -GCaMP6f (9.0 × 10 12 vector genomes ml −1 ), AAV-flex-ChR2-mCherry (3.8 × 10 12 vector genomes ml −1 ) and AAV-CMV-Cre (2.2 × 10 10 vector genomes ml −1 ) was injected via a syringe pump at a rate of 0.1 μl min −1 (KDS310; KD Scientific, Massachusetts, USA) to a depth of 300 μm from the cortical surface. The pipette was inserted vertically and maintained in place for 10 min after the injection. The injection was repeated at 1–3 sites within the rostral motor forelimb area or the caudal motor forelimb area. After the pipette was slowly withdrawn, 4% (w v −1 ) agarose L (Nippon Gene, Tokyo, Japan) was placed over the craniotomy, a 4.5-mm-diameter glass coverslip (number 0 thickness; Matsunami Glass, Osaka, Japan) was pressed onto the agarose surface [13] , and the edges were sealed with dental adhesive resin cement. Mice were then returned to their cages. Mice were allowed to recover and to express sufficient doses of GCaMP7 or GCaMP6f and ChR2 proteins for 2–4 weeks before imaging experiments were performed. Lever-pull task Seven AAV- syn -GCaMP7-transduced mice were used for the self-initiated lever-pull task, which was modified from a previous study [13] . In brief, water-deprived mice were trained to pull a lever for a distance of 5 mm over a time period of 400 ms to obtain a 4 μl drop of water. The water delivery was accompanied by a small click from the water valve. The animals were required to leave the lever at its original position and wait >3 s before pulling the lever again to receive the next water drop. Optical SNOC The seven mice injected with AAV- syn -GCaMP7 and trained at the lever-pull task were used for SNOC by two-photon calcium imaging (2pSNOC). Two-photon calcium imaging was conducted using a FV1000-MPE system (Olympus, Tokyo, Japan) and a mode-locked Ti:sapphire laser (MaiTai HP; Spectra Physics, California, USA) at a wavelength of 910 nm. A 690-nm shortpass dichroic mirror (Olympus) was used to separate the excitation laser and the emitted fluorescence. Fluorescence emissions were collected using a GaAsP photomultiplier tube (PMT; Hamamatsu Photonics, Shizuoka, Japan). The laser intensity was adjusted to 5–36 mW to maintain a constant baseline level of fluorescence in the neurons. The imaged field was 128–512 × 128–268 μm (mean, 380 × 199 μm; n =24 fields from seven mice) and the depth of the imaging plane was 162.5±45.2 μm below the cortical surface ( n =24). The frame duration was 216–311 ms (mean, 292 ms, n =24). The fluorescence intensity of multiple neurons on the monitor of the FV1000-MPE was continuously detected with a machine vision camera (Basler, Ahrensburg, Germany) connected to a personal computer, and was analyzed in real time using a custom-developed and -deployed program written with the assistance of the LabVIEW vision module (National Instruments, Texas, USA). A region of interest (ROI) containing a single neuron was specified, and the mean fluorescence intensity of this ROI was continually measured. When the fluorescence intensity of the ROI remained under the manually determined threshold (3–6 s.d. of the baseline fluorescence intensity) for >1 s and then exceeded the threshold, the mouse was rewarded with two 4-μl drops of water from a spout near the mouth. Simultaneous two-photon imaging and ChR2 photostimulation Six mice injected with AAV- syn -GCaMP6f, AAV-flex-ChR2-mCherry and AAV-CMV-Cre were used for the simultaneous two-photon calcium imaging and ChR2 photostimulation experiments. Relatively low-titered AAV-CMV-Cre (2.2 × 10 10 vector genomes ml −1 ) was stochastically transduced to a limited number of neurons, and relatively high-titered AAV-flex-ChR2-mCherry (3.8 × 10 12 vector genomes ml −1 ) was used to enable strong expression of ChR2 in a sparse subset of neurons. The water-deprived mice were acclimatized to the head restraint and delivery of water from the spout under a microscope for 2 days before the start of the photostimulation experiments. Two-photon calcium imaging was performed in the same way as in the 2pSNOC experiments, except that multialkali PMTs were used instead of GaAsP PMTs to prevent photodamage. The imaged field was fixed to 320 × 160 μm ( n =11 from six mice) and the depth of the imaged plane was 128.5±17.5 μm below the cortical surface ( n =11). The frame duration was 294 ms. A blue-light source (cat. no. MBL-H-473, OptoEngine LLC, Utah, USA) was used for photostimulation [21] , [40] and bifurcated 473-nm light-emitting diodes (LEX2-B; BrainVision, Tokyo, Japan) were set in front of both eyes for masking. The frames that included either photostimulation or masking and one subsequent frame were discarded from the analysis. A 480-nm shortpass dichroic mirror (Olympus) was used to separate the excitation blue light and the emitted fluorescence. Offline processing of imaging data Analyses were performed using ImageJ software (version 1.45s; National Institutes of Health, Maryland, USA) and MATLAB software (versions R2010a, R2011b, MathWorks, Massachusetts, USA). Image sequences were corrected for focal plane displacements by applying the ImageJ plug-in, TurboReg [41] . ROIs were manually specified. Averaging the fluorescence of all pixels within each ROI resulted in a raw time series, from which time-averaged background fluorescence measured in unstained blood vessels was subtracted. The detrended relative change in fluorescence (Δ F / F ) was calculated from the subtracted time series using the eighth percentile value from 15 s before to 15 s after each sample time point [12] , [13] . Non-negative deconvolution [23] of each Δ F / F trace was performed using a decay time constant of 1 s and divided by the median absolute deviation of the deconvoluted trace × 1.3826 × 2 (2 σ). A value of 1 was subtracted from these values. Then, if the values were negative, they were set to zero. The final values were defined as ‘activity’. The ROIs whose activity demonstrated skewness >1 were defined as reconstructed neurons [13] . Further analysis was limited to the reconstructed neurons. In the experiments involving simultaneous two-photon calcium imaging and ChR2 photostimulation, the Δ F / F trace without deconvolution was used for analysis because the light stimulation interrupted continuous monitoring of fluorescence and, therefore, precluded deconvolution. The Δ F / F values in interrupted frames were removed from the analysis. For each neuron, the Δ F / F value 588 ms (two frames) after photostimulation was compared with the Δ F / F value 588 ms after masking stimulation using a one-tailed two-sample t -test. If Δ F / F after photostimulation was significantly larger ( P <0.05) than Δ F / F after masking stimulation, the neuron was defined as a photostimuli-responsive neuron. The number of photostimuli-responsive neurons was 14.8±9.7 ( n =11 fields) per field of view (320 × 160 μm) and this accounted for 43.9% of reconstructed neurons. mCherry fluorescence was detected in 4.9±2.2 cells ( n =8 fields in which mCherry fluorescence was recorded) per field of view (320 × 160 μm) by in vivo two-photon imaging and this accounted for 15.0% of reconstructed neurons; thus, neurons without sufficiently strong mCherry fluorescence should have been included in photostimuli-responsive neurons. ChR2-mCherry-expressing neurons out of the focal plane might also play a role in activating photostimuli-responsive neurons. In 90.2% (156/173) of the photostimuli-responsive neurons, the peak fluorescence value on the first trial was more than half of the peak of the mean fluorescence value on all trials. Thus, the photostimulation immediately evoked activity in the photostimuli-responsive neurons, which eliminates the possibility that the light itself gradually affected the neurons and induced conditioned light responses. Definition of lever-related and lever-unrelated neurons Eight hundred and forty reconstructed neurons were categorized according to their association with the lever movement during the pre-conditioning period. The period from 1 s before the onset of the lever-pull movement to 3 s after the lever had returned to the original position was defined as the lever-related period. During the lever-related period, neurons showing activity that was significantly larger ( P <0.05 by one-tailed two-sample t -test) than that outside the lever-related period were defined as lever-related neurons. The remaining neurons were defined as lever-unrelated neurons. Definition of RSI The 5 s after water delivery was defined as the reward-related period. Spontaneous pairwise correlation was the correlation between the activity of two neurons in reward-unrelated periods of the conditioning period. Activity in reward-related periods was excluded from this analysis to remove any effect of reward-related activity and/or behaviours. The neuronal activity in the first 10 min of the conditioning period was used to calculate RSI( t ). Activity in the final 5 min of the conditioning period was excluded to remove any effect of activity gain and reward gain. RSI( t ) was defined as the sum of activity in a 0.33 s bin t s after reward delivery divided by the sum of activity in reward-unrelated periods. If the time bin t was included in the reward-related period, RSI( t ) was defined as the sum of activity in a 0.33 s bin t s after reward delivery divided by the sum of activity t s after reward delivery and activity in reward-unrelated periods. The duration of the time bin was 0.33 s, which was approximately the duration of a single frame. Because the activity calculated by non-negative deconvolution was ≧ 0, RSI( t ) ranged from 0 to 1 by definition. Analysis of licking behaviour Licking behaviour was monitored at 30 Hz with an infrared video camera during the 2pSNOC experiments and by electrophysiological methods during the photostimulation experiments. To quantify the number of licks per second from the video data, an ROI that included the tongue was selected within the movie and the number of times that the mean intensity of the ROI exceeded a threshold (the mean of the maximum and minimum values in a data set) was counted. To quantify the number of licks per second from the electrophysiological data, the electropotential difference between the spout and the head of the mouse was measured and sampled by the FV1000-MPE. The number of times that the electropotential exceeded a threshold (the mean of the maximum and minimum values in a data set) was counted. Statistics Data are presented as mean±s.d. Student’s t -test, the Wilcoxon signed-rank test, the Wilcoxon rank sum test, Spearman’s correlation test, Pearson’s correlation test and χ 2 -test were used for statistical comparisons. Pairwise comparisons were two-tailed unless otherwise noted. Error bars in graphs represent the s.e.m. ANOVA and post-hoc Tukey’s HSD (honestly significant difference) test were used for multiple comparisons. No statistical tests were run to predetermine sample size. Blinding and randomization were not performed. How to cite this article: Hira R. et al. Reward-timing-dependent bidirectional modulation of cortical microcircuits during optical single-neuron operant conditioning. Nat. Commun. 5:5551 doi: 10.1038/ncomms6551 (2014).